Src-dependent impairment of autophagy by oxidative stress in a mouse model of Duchenne muscular dystrophy Duchenne muscular dystrophy (DMD) is a fatal degenerative muscle disease resulting from mutations in the dystrophin gene. Increased oxidative stress and altered Ca 2+ homeostasis are hallmarks of dystrophic muscle. While impaired autophagy has recently been implicated in the disease process, the mechanisms underlying the impairment have not been elucidated. Here we show that nicotinamide adenine dinucleotide phosphatase (Nox2)-induced oxidative stress impairs both autophagy and lysosome formation in mdx mice. Persistent activation of Src kinase leads to activation of the autophagy repressor mammalian target of rapamycin (mTOR) via PI3K/Akt phosphorylation. Inhibition of Nox2 or Src kinase reduces oxidative stress and partially rescues the defective autophagy and lysosome biogenesis. Genetic downregulation of Nox2 activity in the mdx mouse decreases reactive oxygen species (ROS) production, abrogates defective autophagy and rescues histological abnormalities and contractile impairment. Our data highlight mechanisms underlying the pathogenesis of DMD and identify NADPH oxidase and Src kinase as potential therapeutic targets. Duchenne muscular dystrophy (DMD) is the most common X-linked lethal disorder in humans. It is caused by mutations in the dystrophin gene [1] , [2] , resulting in progressive skeletal muscle degeneration and ultimately leading to paralysis and death [3] . While there is intense research focused on gene and cell-based therapy, to date there is no cure for DMD. Pharmacological-based treatments are aimed at controlling the progression of symptoms, buying time until a genetic or cell-based treatment is realized. How dysfunctional pathways in the dystrophic muscle lead to degeneration is still a matter of intense investigation. The characterization of the culprit pathway(s) linking mutations in dystrophin to muscle degeneration will indeed prove critical in the development of new therapeutic approaches in DMD. Increased Nox2 activity [4] , [5] and Src kinase expression [6] , [7] are thought to underlie the increased oxidative stress in muscles of the mdx mouse, a model of DMD [8] . Recently, impaired autophagy and accumulation of dysfunctional organelles have been reported in dystrophic muscle [9] , [10] , [11] , which may underlie muscle degeneration. Because Src kinase can activate Akt via PI3K (Type I) [12] , [13] , [14] leading to a decrease in mammalian target of rapamycin (mTOR)-dependent autophagy [15] , [16] , we surmised that Nox2 and Src are the critical proteins that link oxidative stress to impaired autophagy in mdx skeletal muscle. We found that in dystrophic muscle increased Nox2 activity increases oxidative stress, activates Src kinase and impairs autophagy by regulating the PI3K/Akt/mTOR pathway. Nox2 increases oxidative stress in mdx mice Using either the nonspecific redox probe DCF ( Supplementary Fig. 1a ) or our Nox2-specific reactive oxygen species (ROS) biosensor p47-roGFP [17] ( Fig. 1a ) we found increased Nox2-specific ROS production in mdx skeletal muscle compared with wild type (WT). The increase in ROS was abolished upon inhibition of Nox2 with the Nox2-specific peptide inhibitor gp91 ds ( Fig. 1a , Supplementary Fig. 1a,b ), scavenging either extracellular or intracellular H 2 O 2 ( Fig. 1a ), or incubating with the antioxidant N-acetyl cysteine ( Supplementary Fig. 1c ). In addition, increased Nox2 activity resulted in intracellular oxidative stress as evidenced by oxidation of the glutathione redox potential probe Grx1-roGFP2 ( Fig. 1b ). Mdx skeletal muscle showed an increase in both total and active Rac1 ( Fig. 1c and Supplementary Fig. 1d ), a regulator of Nox2 activity, as well as phosphorylated and total Src kinase ( Fig. 1d and Supplementary Fig. 1e ) protein levels. While the conversion of total Src into active Src (Y416) was significantly higher in mdx , no significant difference in conversion of total Rac1 to active Rac1 was observed. We also found that the active phosphorylated form of p47 phox was significantly higher in mdx , which was blunted upon incubation with gp91 ds or the selective Src inhibitor, PP2 ( Fig. 1e ). No significant difference in total p47 phox expression level was observed. Inhibition of Src and/or Rac1 decreased oxidation of both p47-roGFP ( Fig. 1f ) and the extracellular H 2 O 2 sensor Amplex-Red ( Fig. 1g ) in mdx skeletal muscle. Thus, Src and Rac1 play major roles in enhanced ROS generation through Nox2 in mdx skeletal muscle. 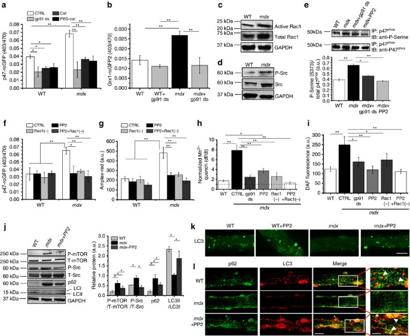Figure 1: Inhibition of Nox2 activity reduces oxidative stress and Src kinase-mediated impaired autophagy. (a) Nox2-specific ROS production was assessed using the Nox2 redox biosensor p47-roGFP redox biosensor Cat: catalase, PEG-Cat: pegylated catalase. (b) Measurement of intracellular glutathione redox potential with Grx1-roGFP2. (c) Analysis of Rac1 and (d) Src. (e) Immunoblot of precipitated p47phoxprobed with an anti-phosphoserine or anti-p47phoxantibody. (f) Nox2-specific intracellular ROS production was measured using p47-roGFP redox biosensor. (g) Extracellular ROS production was assessed using Amplex-red dye. (h) Plasma membrane calcium influx was measured by analysing the Fura-2 fluorescence quench rate upon addition of extracellular Mn2+. (i) Intracellular RNS generation was measured using DAF-FM. Bars represent average±s.e.m. fromn=15 individual fibres for each condition in (a,b,f,g,i,j). Markers of autophagy were analysed in isolated fibres (incubated with or without PP2) from FDBs. (k) Autophagosome formation was analysed using fluorescence microscopy (scale bar=100 μm) and illustrated LC3 localization and autophagosome formation. (l) Confocal microscopy detected p62-LC3 localization in single fibres from FDBs (scale bar=140 and 50 μm for white box areas). All immunoblots were performed with isolated proteins from FDBs and probed with antibodies as indicated. Glyceraldehyde-3-phosphate dehydrogenase (GAPDH) was detected as a loading control. Representative images are shown. Bars represent average ±s.e.m. fromn=3 independent biological experiments. Statistical differences between groups were determined using analysis of variance (ANOVA) with Tukey’spost hoctest. *P<0.05 and **P<0.01. Figure 1: Inhibition of Nox2 activity reduces oxidative stress and Src kinase-mediated impaired autophagy. ( a ) Nox2-specific ROS production was assessed using the Nox2 redox biosensor p47-roGFP redox biosensor Cat: catalase, PEG-Cat: pegylated catalase. ( b ) Measurement of intracellular glutathione redox potential with Grx1-roGFP2. ( c ) Analysis of Rac1 and ( d ) Src. ( e ) Immunoblot of precipitated p47 phox probed with an anti-phosphoserine or anti-p47 phox antibody. ( f ) Nox2-specific intracellular ROS production was measured using p47-roGFP redox biosensor. ( g ) Extracellular ROS production was assessed using Amplex-red dye. ( h ) Plasma membrane calcium influx was measured by analysing the Fura-2 fluorescence quench rate upon addition of extracellular Mn 2+ . ( i ) Intracellular RNS generation was measured using DAF-FM. Bars represent average±s.e.m. from n =15 individual fibres for each condition in ( a , b , f , g , i , j ). Markers of autophagy were analysed in isolated fibres (incubated with or without PP2) from FDBs. ( k ) Autophagosome formation was analysed using fluorescence microscopy (scale bar=100 μm) and illustrated LC3 localization and autophagosome formation. ( l ) Confocal microscopy detected p62-LC3 localization in single fibres from FDBs (scale bar=140 and 50 μm for white box areas). All immunoblots were performed with isolated proteins from FDBs and probed with antibodies as indicated. Glyceraldehyde-3-phosphate dehydrogenase (GAPDH) was detected as a loading control. Representative images are shown. Bars represent average ±s.e.m. from n =3 independent biological experiments. Statistical differences between groups were determined using analysis of variance (ANOVA) with Tukey’s post hoc test. * P <0.05 and ** P <0.01. Full size image Mdx skeletal muscle displays increased sarcolemmal Ca 2+ influx in a redox-dependent manner [4] , [18] . We found that sarcolemmal Ca 2+ influx was increased in quiescent unstretched mdx myofibres, which could be significantly attenuated with gp91 ds, PP2 or Rac1 inhibitors ( Fig. 1h and Supplementary Fig. 2a ). Elevated intracellular Ca 2+ is affiliated with excess reactive nitrogen species (RNS) production in DMD pathology [19] . RNS production, which was significantly higher in myofibres from mdx mice compared with WT, was significantly attenuated by incubation with gp91 ds, PP2 or Rac1 inhibitors ( Fig. 1i and Supplementary Fig. 2b ). These results demonstrate that Src kinase is a key regulator of Nox2 activity, leading to increased oxidative stress and Ca 2+ -dependent RNS production in mdx skeletal muscle. Src kinase regulates mTOR-dependent autophagy in mdx muscle Autophagy is an evolutionarily conserved cellular degradation pathway that contributes to cellular homeostasis and survival by degrading proteins and other cellular constituents. While a role for Src kinase in autophagy impairment has been reported in cancer pathogenesis [12] , the mechanism for impaired autophagy in dystrophic muscle has not been elucidated. Immunoblot analyses showed that phospho-mTOR and phospho-Src levels were significantly increased in mdx skeletal muscle compared with WT ( Fig. 1j ), consistent with a block of autophagy. Accordingly, the levels of the autophagosomal membrane protein, sequestosome-1 (p62), were dramatically increased in mdx skeletal muscle ( Fig. 1j ). Examination of microtubule-associated protein-1 light chain 3 (LC3) showed a prevalence for the lipidated form (LC3II) in WT muscle ( Fig. 1j ), indicating the active formation of autophagic vesicles that were readily detected using confocal microscopy ( Fig. 1k ). Strikingly, mdx muscle was found to have attenuated LC3II levels ( Fig. 1j ) and to be devoid of LC3II-positive vesicles ( Fig. 1k ), indicating dramatic impairment of autophagic flux. Inhibition of Src kinase with PP2 decreased phospho-mTOR and phospho-Src in mdx skeletal muscle, with no change in total protein content ( Fig. 1j ). In addition, a concomitant increase in the ratio of LC3II to LC3I and a decrease in p62 protein levels were observed upon Src inhibition ( Fig. 1j ), providing further evidence for Src-dependent regulation of autophagic flux in mdx skeletal muscle. Importantly, inhibition of Src kinase restored the formation of LC3II-positive autophagic vesicles ( Fig. 1k ). p62, a marker of protein turnover, binds with LC3 and polyubiquitylated proteins, serving as a cargo receptor for the autolysosome degradation process [20] . Immunofluorescence analysis showed a marked decrease in p62 and autophagosome (LC3II) fusion (p62-LC3-positive puncta, yellow), a crucial event in autophagosome clearance, in mdx muscle compared with WT, which was dramatically rescued upon PP2 incubation ( Fig. 1l ). Together, these data suggest that activated Src kinase leads to a block of autophagy in mdx skeletal muscle. Nox2/Src inhibition rescues autophagy in mdx mice A rescue of autophagy induction obtained by inhibiting Src indicated that autophagy is not inherently compromised in mdx muscle. Thus, we investigated the potential downstream signalling pathway associated with autophagy blockage in order to identify possible therapeutic targets. Because the PI3K (type I)/Akt/mTOR/p70S6K axis is a primary regulatory pathway by which autophagy is suppressed, we asked whether impaired autophagy was dependent upon the exuberant activation of Nox2 in mdx muscle. Inhibition of Nox2 with gp91 ds reduced phosphorylation of Src (Y416), PI3K (Y458), Akt (T308) and mTOR (S2448; Fig. 2a ). Likewise, the level of phospho-S6 ribosomal protein (S235/236), a substrate of p70S6K and an indicator of p70S6K activity, also decreased ( Fig. 2a ). No significant changes were observed in WT muscle for any of these signalling molecules ( Fig. 2a ). Given that Nox2 inhibition decreased the phosphorylation of mTOR in mdx muscle, we then investigated autophagic flux. We found a highly significant decrease in p62-LC3 colocalization (yellow puncta) in flexor digitorum brevis (FDB) muscles from mdx mice compared with WT mice ( Fig. 2b ). Inhibition of Nox2 showed a marked recovery in p62-LC3 localization in mdx myofibres ( Fig. 2b ) in conjunction with a higher conversion of LC3I to LC3II, as well as a decrease in p62 protein levels in mdx muscle ( Fig. 2c ). Together, these results demonstrate that inhibition of the Nox2/Src cycle induces mTOR-dependent autophagy. 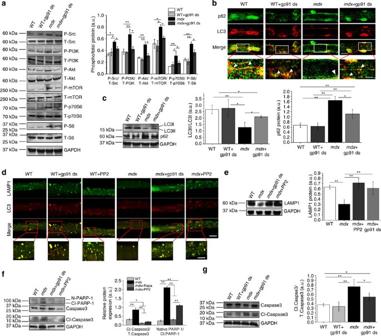Figure 2: Inhibition of Nox2 and Src kinase induces autophagy and prevents cell degeneration in mdx mice via the PI3K/Akt/mTOR pathway. (a) FDB lysates were analysed using immunoblotting with antibodies as indicated. (b) Confocal microscopy shows the effect of Nox2 inhibition on p62-LC3 localization in single FDB fibres. Representative images of independent biological experiments (n=3) are shown (scale bar=100 and 35 μm for white box areas). (c) Autophagic flux was analysed by immunoblotting with anti-LC3B and anti-p62 antibodies. (d) Effect of gp91 ds and PP2 on LC3-LAMP1 colocalization was analysed using confocal microscopy. Representative images from independent biological experiments (n=3) are shown (scale bar=140 and 40 μm for red box areas). (e) Immunoblot analysis of LAMP1, (f) PARP-1 and caspase3 activity. (g) Immunoblot of Caspase3 activity. All immunoblots were performed with isolated proteins from FDBs and probed with antibodies as indicated. GAPDH was detected as a loading control. Representative images are shown. Bars represent average ±s.e.m. fromn=3 independent biological experiments. Statistical differences between groups were determined using ANOVA with Tukey’spost hoctest. *P<0.05 and **P<0.01. Figure 2: Inhibition of Nox2 and Src kinase induces autophagy and prevents cell degeneration in mdx mice via the PI3K/Akt/mTOR pathway. ( a ) FDB lysates were analysed using immunoblotting with antibodies as indicated. ( b ) Confocal microscopy shows the effect of Nox2 inhibition on p62-LC3 localization in single FDB fibres. Representative images of independent biological experiments ( n =3) are shown (scale bar=100 and 35 μm for white box areas). ( c ) Autophagic flux was analysed by immunoblotting with anti-LC3B and anti-p62 antibodies. ( d ) Effect of gp91 ds and PP2 on LC3-LAMP1 colocalization was analysed using confocal microscopy. Representative images from independent biological experiments ( n =3) are shown (scale bar=140 and 40 μm for red box areas). ( e ) Immunoblot analysis of LAMP1, ( f ) PARP-1 and caspase3 activity. ( g ) Immunoblot of Caspase3 activity. All immunoblots were performed with isolated proteins from FDBs and probed with antibodies as indicated. GAPDH was detected as a loading control. Representative images are shown. Bars represent average ±s.e.m. from n =3 independent biological experiments. Statistical differences between groups were determined using ANOVA with Tukey’s post hoc test. * P <0.05 and ** P <0.01. Full size image Since autophagic flux appears to be suppressed in mdx muscle, we investigated whether there was an alteration in autophagosome formation. Colocalization of LC3 and LAMP1 was observed in WT myofibres, with no significant change upon inhibition of Nox2 or Src ( Fig. 2d ). Mdx myofibres showed a highly significant decrease in LC3-LAMP1-positive puncta, which were increased upon inhibition of either Nox2 or Src ( Fig. 2d ), thus confirming a blockage in autophagosome formation. We also observed a significant decrease in LAMP1 expression in mdx myofibres compared with WT, which was markedly restored upon inhibition of Nox2 or Src kinase ( Fig. 2e ). qPCR analysis of mRNA extracted from WT and mdx FDBs showed around a 33% decrease in LAMP1 transcript in mdx compared with WT ( Supplementary Fig. 3 ). These results suggest that increased oxidative stress may be a key regulatory factor of lysosomal maturation in mdx skeletal muscle. Impaired autophagy is associated with aggregation of proteins and other cellular constituents, eventually leading to cell degeneration. Therefore, we investigated whether impaired autophagy in mdx muscle could lead to cell death. We found a marked increase in the apoptotic markers, poly [ADP-ribose] polymerase 1 (PARP-1) and cleaved caspase3, in mdx muscle compared with WT, which was significantly reduced upon inhibition of Src kinase activity ( Fig. 2f ). Mdx fibres incubated with rapamycin (an mTOR inhibitor) also showed a decrease in the cleavage of apoptotic markers ( Fig. 2f ). Inhibition of Nox2 activity led to a significant decrease in caspase3 cleavage ( Fig. 2g ). Taken together, our data demonstrate that the Nox2 complex plays a major role in impaired autophagy and muscle degeneration in mdx mice. Inhibition of Nox2 activity may lead to a decrease in cell degeneration by restoring autophagy. Decreased Nox2 ROS and rescued autophagy in p47 −/− - mdx mice Having established Nox2 and Src kinase as the key upstream regulators of impaired autophagy in mdx skeletal muscle using pharmacological inhibitors, we next took a genetic approach to corroborate our findings. Genetic knockout of p47 phox attenuates ROS generation in skeletal muscle [17] . Therefore, we hypothesized that genetic abrogation of p47 phox function in mdx mice would be beneficial against oxidative stress-induced damage. In muscle from mice deficient in p47 phox and dystrophin (p47 −/− - mdx ) we found a highly significant reduction in ROS generation and Ca 2+ influx ( Fig. 3a,b ), as well as a marked decrease in phosphorylation of Src kinase ( Fig. 3c ) compared with mdx . Reduced phosphorylation of mTOR, a significant increase in LC3I to LC3II conversion, and a concomitant decrease in p62 expression levels were evident in FDBs from p47 −/− - mdx mice compared with mdx ( Fig. 3d ), indicating enhanced autophagic flux in p47 −/− - mdx compared with mdx . Treatment of myofibres with rapamycin increased LC3II to LC3I ratios and decreased p62 and phospho-mTOR levels in mdx myofibres ( Fig. 3d ). We also found a rescue in LAMP1 protein expression and fusion of LC3 and LAMP1-positive vesicles in p47 −/− - mdx mice compared with mdx mice ( Fig. 3e ). Rescue of autophagy was also observed in tibialis anterior (TA), diaphragm (Dia) and soleus skeletal muscles of p47 −/− - mdx mice ( Supplementary Fig. 4a–c ). Thus, inhibition of Nox2 activity rescues mdx muscle from oxidative stress and subsequently maintains the homeostasis of the autophagic machinery. 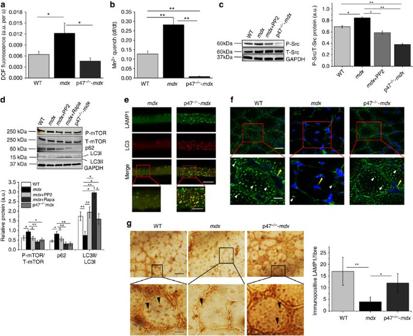Figure 3: Genetic deletion of p47phoxdecreases oxidative stress and induces activation of autophagy inmdxmice. (a) Intracellular ROS production was assessed using DCFH-DA. (b) Plasma membrane calcium influx was measured by analysing the quench of Fura-2 fluorescence upon addition of extracellular Mn2+. (a,b) Were conducted in enzymatically digested single FDBs from WT,mdxand p47−/−-mdxmice. Bars represent average±s.e.m. fromn=15 individual fibres for each condition. (c) Immunoblot analysis of Src protein with anti-P-Src or anti-Src antibodies. (d) Autophagy marker proteins were analysed by immunoblotting with antibodies as indicated (c) and (d) were conducted in enzymatically isolated fibres from FDBs of WT,mdxand p47−/−-mdxmice. Representative images are shown. GAPDH was detected as a loading control. Bars represent average±s.e.m. fromn=3 independent biological experiments. (e) LC3-LAMP1 colocalization in single FDBs frommdxand p47−/−-mdxmice was analysed using confocal microscopy. Representative images fromn=3 independent biological experiments are shown (scale bar=100 and 40 μm for red box areas). (f) Immunofluorescence assay to detect lysosomes (LAMP1) in TA muscle from WT,mdxand p47−/−-mdxmice. White arrows indicate lysosome and yellow arrows indicate nucleus. (g) Immunohistochemistry to detect lysosome (LAMP1) in TA muscle from WT,mdxand p47−/−-mdxmice. Black arrows indicate LAMP1 positive (brown) structures. Histogram plot quantifying the number of immunopositive LAMP1 structures per fibre. Representative images fromn=3 independent biological experiments are shown. Scale bar represents 100 μm forfand 140 μm forg. Statistical differences between groups were determined using ANOVA with Tukey’spost hoctest. *P<0.05 and **P<0.01. Figure 3: Genetic deletion of p47 phox decreases oxidative stress and induces activation of autophagy in mdx mice. ( a ) Intracellular ROS production was assessed using DCFH-DA. ( b ) Plasma membrane calcium influx was measured by analysing the quench of Fura-2 fluorescence upon addition of extracellular Mn 2+ . ( a , b ) Were conducted in enzymatically digested single FDBs from WT, mdx and p47 −/− - mdx mice. Bars represent average±s.e.m. from n =15 individual fibres for each condition. ( c ) Immunoblot analysis of Src protein with anti-P-Src or anti-Src antibodies. ( d ) Autophagy marker proteins were analysed by immunoblotting with antibodies as indicated ( c ) and ( d ) were conducted in enzymatically isolated fibres from FDBs of WT, mdx and p47 −/− - mdx mice. Representative images are shown. GAPDH was detected as a loading control. Bars represent average±s.e.m. from n =3 independent biological experiments. ( e ) LC3-LAMP1 colocalization in single FDBs from mdx and p47 −/− - mdx mice was analysed using confocal microscopy. Representative images from n =3 independent biological experiments are shown (scale bar=100 and 40 μm for red box areas). ( f ) Immunofluorescence assay to detect lysosomes (LAMP1) in TA muscle from WT, mdx and p47 −/− - mdx mice. White arrows indicate lysosome and yellow arrows indicate nucleus. ( g ) Immunohistochemistry to detect lysosome (LAMP1) in TA muscle from WT, mdx and p47 −/− - mdx mice. Black arrows indicate LAMP1 positive (brown) structures. Histogram plot quantifying the number of immunopositive LAMP1 structures per fibre. Representative images from n =3 independent biological experiments are shown. Scale bar represents 100 μm for f and 140 μm for g . Statistical differences between groups were determined using ANOVA with Tukey’s post hoc test. * P <0.05 and ** P <0.01. Full size image p47 −/− - mdx mice show significant rescue in lysosomal biogenesis Because autophagy is a lysosome-dependent process, we next investigated the status of lysosomal biogenesis in mdx muscle. Both immunofluorescence ( Fig. 3f ) and immunohistochemical assays ( Fig. 3g ) showed a marked decrease in lysosome formation in mdx muscle compared with WT, indicating that exuberant activation of Nox2 and Src kinase impairs lysosome biogenesis. Interestingly, analysis of p47 −/− - mdx muscle showed rescue of lysosomal biogenesis compared with mdx ( Fig. 3f,g ) These results identify the lysosomal-autophagy pathway as a critical and reversible point of intersection among pathways that are dysregulated in the cellular pathogenesis of DMD. Improved pathophysiological abnormalities in p47 −/− -mdx Since genetic ablation of p47 phox rescued mdx muscle from excess ROS production, exuberant sarcolemmal Ca 2+ influx and defective autophagy-lysosomal function, we next investigated whether these changes improved the pathological abnormalities and contractile dysfunction of mdx skeletal muscle. Haematoxylin and eosin (H&E) staining revealed decreased cross-sectional area (CSA; 292 versus 470 μm 2 ) and increased centronucleated myofibres (57% versus 5%) in mdx Dia, compared with WT ( Fig. 4a ), both hallmarks of the dystrophic phenotype. Dia muscle from p47 −/− - mdx mice showed a decrease in the number of centronucleated myofibres (30%) and a shift in the CSA (521 μm 2 ) to larger fibres, similar to WT ( Fig. 4a ). TA from mdx mice showed a significant increase in immune cell infiltration compared with WT, which was markedly decreased in p47 −/− - mdx mice ( Fig. 4b ). We found that ablation of p47 phox in mdx skeletal muscle prevented the IIB to IIA fibre-type switch that occurs in mdx skeletal muscle ( Fig. 4c ). In mdx mice, serum creatine kinase (CK) was 37.5-fold higher than WT. There was a trend for a decrease (22.6%) in serum CK activity in p47 −/− - mdx mice compared with mdx ; however, it did not reach statistical significance ( Fig. 4d ). Importantly, we also found that Dia muscle from p47 −/− - mdx mice had greatly improved functional properties compared with Dia from mdx mice ( Fig. 4e ). Both twitch and tetanic forces were significantly lower in mdx Dia compared with WT (41% and 49%, respectively). Genetic downregulation of Nox2 significantly improved both twitch (50%) and tetanic (31%) force productions in the Dia from p47 −/− - mdx compared with mdx . Taken together, our results show that downregulation of the Nox2/Src pathway improves the pathological and functional defects of dystrophic skeletal muscle by upregulating the autophagy-lysosome system. 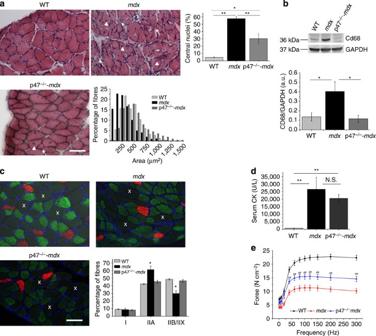Figure 4: Genetic inhibition of Nox2 activity ameliorates pathological and functional phenotypes in dystrophic muscle. (a) Haematoxylin and eosin staining of cross-sections from Dia showing central nuclei (arrow head) and smaller fibres (arrow). (b) Immunoblot analysis of macrophage content (CD68). (c) Immunofluorescent and bright field images of Dia cross-sections showing fibre-type distribution. Type I (red), IIA (green), IIB/IIX ( white x, unstained and viewed from bright field overlay). (d) Serum creatine kinase activity. (e) Force–frequency relationship in Dia muscle strips from WT (black),mdx(red) and p47−/−-mdx(blue) mice. Scale bars represent 55 μm. Fore,#P<0.01 p47−/−-mdxversusmdx.##P<0.01 p47−/−-mdxversus WT andmdx. Mdxwas statistically different than WT at all frequencies of stimulation. Statistical differences between groups were determined using ANOVA with Tukey’spost hoctest. *P<0.05 and **P<0.01. Figure 4: Genetic inhibition of Nox2 activity ameliorates pathological and functional phenotypes in dystrophic muscle. ( a ) Haematoxylin and eosin staining of cross-sections from Dia showing central nuclei (arrow head) and smaller fibres (arrow). ( b ) Immunoblot analysis of macrophage content (CD68). ( c ) Immunofluorescent and bright field images of Dia cross-sections showing fibre-type distribution. Type I (red), IIA (green), IIB/IIX ( white x, unstained and viewed from bright field overlay). ( d ) Serum creatine kinase activity. ( e ) Force–frequency relationship in Dia muscle strips from WT (black), mdx (red) and p47 −/− - mdx (blue) mice. Scale bars represent 55 μm. For e , # P <0.01 p47 −/− - mdx versus mdx. ## P <0.01 p47 −/− - mdx versus WT and mdx. Mdx was statistically different than WT at all frequencies of stimulation. Statistical differences between groups were determined using ANOVA with Tukey’s post hoc test. * P <0.05 and ** P <0.01. Full size image Previous work has reported upregulation of Nox2 content before an increase in immune cell infiltration [4] . The signalling pathways modified by Nox2-dependent ROS, however, have not been identified. Increased activation of mTOR [21] and impaired autophagy have been observed in mdx skeletal muscle [9] , [22] . While treatment of mdx mice with rapamycin (an mTOR inhibitor) [21] or a prolonged low-protein diet [9] were able to reduce muscle inflammation, necrosis and muscle damage, the mechanisms leading to defective autophagy and the potential upstream regulatory pathways were not investigated. In this study we establish, for the first time, a mechanism by which Nox2-specific oxidative stress impairs autophagy, through Src kinase-dependent activation of the PI3K/Akt/mTOR pathway. Furthermore, we discovered that lysosome formation is defective in mdx skeletal muscle ( Fig. 5 ). Proper lysosome formation is necessary for recycling of molecules and nutrients as well as to get rid of the cells of unwanted or damaged organelles. The severe decrease in lysosomal biogenesis in mdx mice may lead to the failure in starvation-dependent activation of autophagy in mdx mice [9] . Pharmacological or genetic inhibition of Nox2 reactivated autophagy, rescued lysosomal biogenesis and rescued the pathological as well as the physiological phenotype of dystrophic skeletal muscle. Our data indicate that pharmacological or genetic inhibition of Nox2 or Src kinase may prove to be beneficial therapeutic targets for the treatment of DMD. 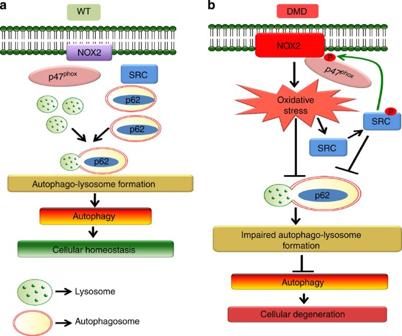Figure 5: Proposed mechanism for Nox2/Src-dependent impaired autophagy in DMD pathology. (a) Autophagic machinery functions properly in WT condition through autophagosome and lysosome fusion, maintaining cellular homeostasis. (b) Upregulation of Nox2/Src activity prevents autophagolysosome formation, impairing autophagy and leading to cellular degeneration in DMD. Figure 5: Proposed mechanism for Nox2/Src-dependent impaired autophagy in DMD pathology. ( a ) Autophagic machinery functions properly in WT condition through autophagosome and lysosome fusion, maintaining cellular homeostasis. ( b ) Upregulation of Nox2/Src activity prevents autophagolysosome formation, impairing autophagy and leading to cellular degeneration in DMD. Full size image Using our targeted redox biosensor p47-roGFP [17] , we established that the Nox2 complex is a significant source of oxidative stress in mdx skeletal muscle. Nox2-dependent ROS production enhanced Ca 2+ influx and generation of RNS, as well as activated Src kinase, which in turn leads to further activation of Nox2 via p47 phox phosphorylation. Although we cannot exclude the involvement of other ROS sources (that is, the mitochondria), inhibition of the Nox2 complex and Src kinase significantly reduced oxidative stress in mdx muscle. Autophagy is a dynamic cellular pathway involved in maintenance of cellular homeostasis by degradation of misfolded/toxic proteins and other damaged cellular constituents [23] . Impaired autophagic flux is detrimental to skeletal muscle and plays a major role in the pathology of several skeletal muscle disorders [11] , [24] . We found a significant enhancement in phosphorylated Src and reduction in the lipidated form of LC3 (LC3II) in muscle fibres from mdx mice. Reduction of LC3II protein and LC3-positive puncta was accompanied by enhanced presence of phosphorylated mTOR and increased levels of p62, all of which support a decrease in autophagic flux in mdx skeletal muscle. Inhibition of either Nox2 or Src kinase in mdx skeletal muscle was able to inhibit the PI3K/Akt/mTOR pathway, decrease p62 levels and restore LC3II levels. Inhibition of autophagy can lead to degeneration of skeletal muscle [25] . In agreement with previous reports, we found increased apoptosis in muscle fibres from mdx mice compared with WT mice, which could be partially attenuated by inhibition of Nox2 or Src kinase. These findings support our hypothesis that Nox2 and Src kinase are the key regulatory factors in defective autophagic machinery in mdx muscle. Our data appear to be contrary to evidence in the literature that support a role for ROS-induced autophagy, for review see refs 26 , 27 . Huang et al. [28] report that Nox2-derived ROS is important for autophagy induction in phagocytic cells while here we show that Nox2 ROS impairs autophagy. This dichotomy may lie in the spatial and temporal production of ROS. ROS participate in cellular signalling; however, when produced at high levels or for extended periods of time they can cause irreversible oxidative damage. Dystrophic skeletal muscle is under constant oxidative stress. In addition, the subcellular localization of Nox2 with Src kinase in caveolae within the skeletal muscle sarcolemma [4] , [6] may provide a spatially privileged communication, allowing Nox2-dependent ROS to activate Src and the PI3K/Akt/mTOR pathway and thereby inhibit autophagy. Late autophagy is marked by autophagosome coalescence and fusion with lysosomes to form autolysosomes. It has been reported that elevated oxidative stress is associated with decreased LAMP1 expression and impaired lysosomal maturation [29] . Muscle fibres from mdx mice contain a marked decrease in LC3/LAMP1 autolysosome-positive structures and a significant reduction in the expression of LAMP1, which can be restored with pharmacological or genetic inhibition of Nox2-specific oxidative stress. Further, we saw a significant decrease in lysosome coalescence in mdx muscle. Lysosomes have long been identified as participating in signalling pathways that sense nutrient deprivation and facilitate energy metabolism by inducing autophagy in response to starvation [30] . Clementi and colleagues [9] have reported a failure in the activation of autophagy in mdx mice in response to starvation. In this study, we found severe damage in lysosomal biogenesis in mdx mice, suggesting that lack of lysosome formation may lead to failure of starvation-dependent activation of autophagy in mdx mice. These findings indicate that DMD may be characterized as a lysosomal dysfunctional disorder. Transcriptional behaviour and functional integrity of most of the lysosomal genes are regulated by transcription factor EB (TFEB) [31] . While oxidative stress has been suggested to downregulate functional activity of TFEB and lysosomal activity [32] , the specific mechanisms of action are yet to be established. We are currently investigating the regulatory mechanisms of TFEB in transcription of LAMP1 in mdx skeletal muscle. To investigate the role of Nox2/Src kinase-dependent impairment of autophagy in the pathophysiology of DMD, we assessed several histopathological markers and muscle function upon genetic downregulation of Nox2 activity. In the mdx mouse muscle, infiltration of immune cells is recognized by 3–4 weeks of age, followed by massive degeneration/necrosis, elevated serum CK activity and replacement of muscle with fibrosis and fatty tissue at around 12 weeks of age. In our studies we observed significant improvement of the pathophysiological phenotype of Dia muscle from young (4–6 weeks) p47 −/− - mdx mice, an age before replacement of muscle fibres with fibrotic and fatty tissues, as evidenced by prevention of IIB to IIA fibre-type switch, maintenance of CSA and percent fibres with central nuclei, and reduced immune cell infiltration. Consistent with previous reports, we found a significant increase in serum CK levels in mdx mice compared with WT mice. However, p47 −/− - mdx mice did not show a significant reduction in serum CK levels compared with mdx mice. Creatine kinase can be released from the muscle in response to fibre damage, degeneration/regeneration or necrosis. We found a significant decrease in apoptosis in muscle from p47 −/− - mdx mice and protection against a decline in force production in Dia muscle; thus, the elevated serum CK levels in the p47 −/− - mdx mice may be because of some persistent ongoing degeneration/regeneration. In the mdx mouse the Dia is the most severely dystrophic skeletal muscle and best represents the progression of the human disease. Since respiratory failure is a leading cause of death in DMD, rescuing the functional deficits in dystrophic Dia will improve respiratory function and therefore quality of life for patients suffering from DMD. In conclusion, this study demonstrates the presence of a Nox2/Src kinase-dependent impairment of autophagy in mdx skeletal muscle. Both pharmacological and genetic inhibition of Nox2 or Src kinase led to restoration of the autophagic machinery and improvement of the pathophysiological phenotype. As Nox2 and Src kinase are upregulated early in the progression of the disease, before muscle damage and inflammation, Nox2/Src may prove to be beneficial therapeutic targets for the treatment of DMD. Targeting Src kinase is of particular interest, as Src kinase inhibitors are currently in Phase II clinical trials for the treatment of certain types of cancer. Additional preclinical studies are currently underway in our laboratory to assess the efficacy of in vivo Src inhibitors on the pathophysiology of dystrophic muscle. Chemical reagents and antibodies PP2 was purchased from Calbiochem. Rapamycin, pegylated-catalase, catalase, N-Acetyl Cysteine and ECM gel (from Engelbreth–Holm–Swarm murine sarcoma) were purchased from Sigma-Aldrich. Fura-2/AM, DAF-FM, Amplex-red and DCFH-DA (6-carboxy-2′,7′-dichlorodihydrofluorescein diacetate) were from Invitrogen. The Nox-specific peptide inhibitor gp91 ds was from Biosynthesis, Lewisville, TX, USA. Anti-Src, anti-P-Src, anti-PI3K, anti-P-PI3K, anti-Akt, anti-P-Akt, anti-mTOR, anti-P-mTOR, anti-p70S6K, anti-P-p70S6K, anti-S6, anti-P-S6, anti-caspase3, anti-Cleaved-caspase3, anti-LC3B, anti-PARP-1 and anti-LAMP1 antibodies were from Cell Signalling Technology. Anti-glyceraldehyde-3-phosphate dehydrogenase, anti-active Rac1, anti-p47 phox and anti-P-serine were purchased from Millipore. Anti-Type I (BA-F8) and anti-Type IIA (SC-71) were purchased from Developmental Studies Hybridoma Bank (DSHB). IgG1 and IgG2b isotype-specific secondary antibodies were purchased from Invitrogen. Anti-p62 and Protein G PLUS-Agarose were from Santa Cruz Biotechnologies. Anti-Rac1 was from Abcam. ODYSSEY secondary antibodies for western blot (anti-mouse 680 , anti-mouse 800 , anti-rabbit 680 , anti-rabbit 800 and anti-goat 800 ) were purchased from LI-COR Biosciences. Secondary antibodies for immunofluorescence (Alexa Fluor 488 Chicken-anti-mouse and Alexa Fluor 594 Donkey-anti-rabbit) were purchased from Invitrogen. DMEM was from Gibco, heat-inactivated fetal bovine serum was purchased from Atlanta Biologicals. Ninety-six-well plates were from Costar, X-tremeGENE HP DNA Transfection Reagent and Collagenase A were from Roche Applied Science. Detailed information about antibodies and dilution can be found in Supplementary Table 1 . Generation of p47 phox -dystrophin double knockout animals Male homozygous mice lacking p47 phox (B6(Cg)- Ncf1 m1J /J, JaxMice) were crossed with female homozygous dystrophic deficient mice C57BL/10ScSn- Dmd mdx /J, JaxMice) to generate p47 phox+/− -dystrophin +/− mice. Male and female siblings were mated to generate p47 phox−/− -dystrophin −/− female mice. Female p47 phox−/− -dystrophin −/− mice were back-crossed with p47 phox−/− males to generate p47 phox−/− -dystrophin +/− females. These p47 phox−/− -dystrophin +/− female mice were back-crossed with p47 phox−/− males for at least six generations to obtain mice on a C57BL6/J background. Isolation of FDB fibres and treatment Mice were deeply anaesthetized by isoflurane (2%) inhalation and killed by rapid cervical dislocation in accordance with the National Institutes of Health guidelines and approved by the Institutional Animal Care and Use Committee of Baylor College of Medicine. FDB muscles were surgically isolated and incubated in minimal essential media containing 0.1% gentamycin and 0.4% Collagenase A at 37 °C for 1.5–2.0 h. To release single fibres, FDB muscles were then triturated gently in serum containing media (10%, Atlanta Biologicals) without collagenase and incubated in 5% CO 2 at 37 °C until used, typically 12–36 h later. All other muscles were rapidly frozen in liquid nitrogen and stored at −80 °C until used. For western blotting and immunostaining, fibres were treated with PP2 (0.2 μM) or gp91 ds (5 μM) at 37 °C for 24 h. For all other experiments, fibres were incubated with PP2 (0.2 μM), gp91 ds (5 μM) or Rac1 inhibitor (50 μM) at 37 °C for 2 h. ROS measurements Enzymatically digested single FDBs were seeded on 96-well plates for either intracellular (DCFH-DA) or extracellular (Amplex-red) ROS measurements. DCF fluorescence was excited at 480 nm via a Sutter Lamda DG-5 Ultra high-speed wavelength switcher, and emission intensity was collected at 510 nm at a rate of 0.1 Hz. Amplex-red dye was excited at 550 nm via a Sutter Lamda DG-5 Ultra-high speed wavelength switcher and emission intensity was collected at 590 nm at a rate of 0.1 Hz. For assessment of Nox2 activity and glutathione redox potential (oxidative stress), FDBs were electroporated with either p47-roGFP or Grx1-roGFP2, respectively, and fluorescence ratios quantified as previously described [17] , [33] . Assessment of Ca 2+ influx by Mn 2+ quench and RNS measurement Calcium influx was assessed using the Mn 2+ quench of Fura-2 fluorescence as previously reported [3] , [34] . RNS was measured using DAF-FM dye. Excitation was at 488 nm and emission was captured with a linear detector after passing through a 495- to 555-nm band pass filter. Western blotting Lysates from either enzymatically digested FDBs or whole tissue (Dia, TA, soleus and extensor digitorum longus) were extracted and quantified with the bicinchoninic acid protein assay kit (Pierce, Rockford, IL, USA), using bovine serum albumin as standard. Lysates were separated via SDS–PAGE and then transferred to polyvinyldifluoride membranes. Blots were incubated in blocking buffer (5%, w/v, dried skimmed milk in Tris-buffered saline, pH 7.4, and 0.2% Tween 20, TBST) followed by overnight incubation with appropriate antibodies diluted in blocking buffer (5% bovine serum albumin in TBST). Blots were then exposed to the IRDye Secondary Antibodies (LI-COR) diluted in TBST for 60 min at room temperature and washed again. Blots were detected using LI-COr Odyssey Infrared Imaging System and analysed using the ImageJ software. Representative uncropped blots are shown in Supplementary Fig. 5 . Immunoprecipitation of p47 phox For p47 phox immunoprecipitation, enzymatically digested FDB fibres were incubated in the absence and presence of gp91 ds or PP2 and the cytosolic fraction (100 μg protein) was transferred to microcentrifuge tubes, and anti-p47 phox antibody (15 μg) was added and incubated for 60 min at 4 °C. Agarose conjugate (30 μl, Protein G PLUS-Agarose) was added and incubated (60 min, 4 °C). Samples were centrifuged, and the supernatant was subjected to immunoblotting and probed with anti-phosphoserine antibody and anti-p47 phox antibodies. Assessment of autophagy by immunostaining FDB muscles were removed immediately after killing and cultured overnight with or without treatment. On the day of experiments, fibres were plated on ECM gel from Engelbreth–Holm–Swarm murine sarcoma (Sigma, St Louis, MO, USA)-coated glass-bottom culture dishes for 1 h. Fibres were then fixed with 4% paraformaldehyde in 0.1 M phosphate buffered saline (PBS) for 15 min. Fibres were blocked with blocking reagent (0.1% saponin, 8% goat serum in PBS) for 1 h. The fibres were then permeabilized with 0.1% triton, incubated with primary antibody (LC3 and LAMP1) overnight at 4 °C, washed, incubated with secondary antibodies for 2 h and washed again before microscopy. Histology and serum CK activity Serial sections of 12-μm thickness were cut from the mid-belly region of Dia and TA muscles on a refrigerated cryostat (Shandon Cryotome E, Thermo) at −20 °C. Sections were stained with H&E and Masson’s Trichrome. Digitized images (8 bit) of muscle sections were acquired with a CCD camera (Digital Sight DS-Fi1, Nikon) attached to an upright microscope (Nikon Eclipse 80i). Images were analysed with NIS Elements Br software (Nikon) where the mean CSA of muscle fibres was calculated by interactive determination of the circumference of at least 200 adjacent cells from the centre of every muscle section examined. Percentage of central nuclei was determined from at least 200 fibres from at least three mice of each genotype. For serum CK activity, blood was drawn from the saphenous vein, serum-separated and CK activity measured on a Cobas Integra 400/800 analyzer (Roche). Immunofluorescence and immunohistochemistry Serial sections of 6- to 12-μm thickness were fixed with cold methanol for 20 min. For immunofluorescence, frozen tissue sections were incubated overnight with appropriate antibodies in a humid box at 4 °C followed by incubation with appropriate secondary antibody (1:300) for 3 h. Slides were then mounted with vectashield containing 4′,6-diamidino-2-phenylindole (H-1200). For the immunohistochemistry, frozen sections were incubated with 0.3% H 2 O 2 solution in PBS at room temperature for 20 min to quench endogenous peroxidase activity and incubated with the primary antibody overnight at 4 °C in a humid box. The sections were then subjected to the secondary antibody from the VECTASTAIN Elite ABC kit (Vector Lab) according to the manufacturer’s instructions. The slides were developed with DAB substrate kit (SK-4100). Real-time PCR Total RNA was extracted from FDBs of WT and mdx mice by using a miRNeasy Mini kit (Qiagen), and 1 mg of total RNA was used to synthesize cDNA using Quantitect reverse transcription kit (Qiagen). Real-time quantitative RT–PCR on cDNAs was carried out with the iTaq Universal SYBR Green Supermix (Bio-Rad) using the CFX96 real-time PCR detection system (Bio-Rad) with the following conditions: 95 °C, 5 min (95 °C, 10 s; 60 °C, 10 s; 72 °C, 15 s) × 40. For expression studies, the qRT–PCR results were normalized against an internal control (Cyclophillin). Oligonucleotide sequences were: Lamp1-F (5′-CCTACGAGACTGCGAATGGT-3′) Lamp1-R (5′-CCACAAGAACTGCCATTTTTC-3′) Cyclophilin-F (5′-GGCAAATGCTGGACCAAACACAA-3′) Cyclophilin-R (5′-GTAAAATGCCCGCAAGTCAAAAG-3′). Ex vivo force measurements Dia muscle was dissected from mice and one end tied to a fixed hook and the other to a force transducer (F30, Harvard Apparatus) using silk suture (4-0) in a physiological saline solution continuously gassed with 95% O 2 –5% CO 2 at 30 °C. Contractile properties were assessed by passing a current between two platinum electrodes at supramaximal voltage (PanLab LE 12406, Harvard Apparatus) with pulse and train durations of 0.25 and 400 ms, respectively. Muscle length was adjusted to elicit maximum twitch force (optimal length, Lo) and the muscle was allowed a 15-min equilibration period. To define the force–frequency characteristic force was measured at stimulation frequencies of 1, 5, 10, 20, 40, 60, 80, 120, 150 and 200 Hz every 1 min. At the end of the contractile protocol, muscle length was measured using a hand-held electronic caliper, fibre bundles removed from the organ bath and trimmed of excess bone and connective tissue, blotted dry and weighed. Muscle weight and Lo were used to estimate CSA and absolute forces expressed as N cm −2 (ref. 35 ). Data analysis Data are reported as mean±s.e.m., unless otherwise specified. Statistical differences between groups were determined using analysis of variance with Tukey’s post hoc test. Statistical analysis was performed in Origin Pro (OriginLab Corporation, Northhampton, MA, USA) with a significance level of * P <0.05 and ** P <0.01. Colocalization analysis in single fibres was performed using ImageJ. How to cite this article: Pal, R. et al. Src-dependent impairment of autophagy by oxidative stress in a mouse model of Duchenne muscular dystrophy. Nat. Commun. 5:4425 doi: 10.1038/ncomms5425 (2014). The content is solely the responsibility of the authors and does not necessarily represent the official views of the National Institutes of Health.